Reductive glutamine metabolism is a function of the α-ketoglutarate to citrate ratio in cells Reductively metabolized glutamine is a major cellular carbon source for fatty acid synthesis during hypoxia or when mitochondrial respiration is impaired. Yet, a mechanistic understanding of what determines reductive metabolism is missing. Here we identify several cellular conditions where the α-ketoglutarate/citrate ratio is changed due to an altered acetyl-CoA to citrate conversion, and demonstrate that reductive glutamine metabolism is initiated in response to perturbations that result in an increase in the α-ketoglutarate/citrate ratio. Thus, targeting reductive glutamine conversion for a therapeutic benefit might require distinct modulations of metabolite concentrations rather than targeting the upstream signalling, which only indirectly affects the process. Uncontrolled cell proliferation associated with cancer necessitates metabolic alterations to support rapid cell growth; hence, understanding these changes is of critical importance in identifying new and promising cancer therapies [1] , [2] . Although substantial progress has been made in elucidating how altered signalling events promote uncontrolled proliferation in cancer, our knowledge regarding the metabolic rearrangements that provide building blocks for biomass, ATP and generation of reducing equivalents remains limited [3] , [4] . Recently, we and other groups identified reductively metabolized glutamine as the major carbon source of fatty acid synthesis during hypoxia and impaired respiration [5] , [6] , [7] , [8] . Moreover, this switch in carbon source selection was shown to be of particular importance for sustaining rapid cell proliferation [5] , [7] . Both hypoxia and the loss of the Von-Hippel Lindau gene ( VHL ) [9] , [10] promote reductive glutamine metabolism, whereas inhibition of pyruvate dehydrogenase kinase isoform 1 (PDK1), a target of the VHL–hypoxia-inducible factor 1α axis [11] , [12] , also decreases reductive glutamine utilization in various cell systems [5] , [7] . In addition, reductive glutamine utilization is activated during impaired respiration, thereby raising the possibility that alterations in NAD + /NADH metabolism might be involved [6] . However, a mechanistic understanding of how hypoxia, respiratory impairment and expression changes in VHL and PDK1 all converge to impact reductive glutamine metabolism is lacking. As a result, the prediction of how other environmental, genetic or pharmacological interventions might trigger reductive glutamine utilization is not possible. In this study we aim to identify how the switch to reductive glutamine utilization is controlled in cells. To this end we systematically measure changes in metabolite levels and metabolic flux contributions in cancer cell lines, following various cellular perturbations, and examine the impact of these changes on reductive glutamine metabolism. We find that reductive glutamine metabolism is a general phenomenon that occurs in response to any intervention that increases the α-ketoglutarate/citrate ratio. Specifically, changes in this ratio are predicted to increase reductive glutamine metabolism by mass action. Furthermore, in most conditions tested, a decrease in acetyl-CoA (AcCoA) to citrate conversion, triggered by one of at least two different mechanisms, is an event responsible for the alteration in the α-ketoglutarate/citrate ratio, suggesting this as a key node in determining reductive glutamine metabolism. Oxidative and reductive glutamine metabolism In mammalian cells, glutamine can be an important contributor of carbon to the tricarboxylic acid (TCA) cycle [13] , [14] , where it can be metabolized in the oxidative or reductive direction [5] , [6] . Reductive glutamine metabolism involves the conversion of α-ketoglutarate to citrate and acts as a carbon source to fuel fatty acid synthesis ( Fig. 1a ). In oxidative glutamine metabolism, α-ketoglutarate is oxidized to succinate for the eventual conversion to citrate by the TCA cycle. Interconversion of citrate and isocitrate is necessary for the TCA cycle to operate in either direction; this reaction is often found close to equilibrium such that isocitrate is maintained at ~6.5% of the citrate concentration [15] . We experimentally validated the equilibrium assumption for the culture conditions and treatments tested here, and found the isocitrate concentration to be 4.1±0.79% of the citrate concentration under standard culture condition and 5.3±0.85% of the citrate concentration following metformin treatment. Therefore, to simplify our analysis we focused our measurements on citrate as the more abundant metabolite. As α-ketoglutarate and citrate levels represent the substrate or product in key reactions of reductive versus oxidative glutamine metabolism, their levels are predicted to be critical parameters in determining the reaction direction. Although both metabolites are present in the cytosol and the mitochondria, we analysed the total pool size because of the lack of established methods to quantitatively separate the two pools. Furthermore, we decided to specifically focus on the reductive glutamine contribution instead of the reductive net flux, because net fluxes per se are also a function of growth rate [16] . As many of the perturbations used in this study influence cell growth, it is impossible to control for secondary effects on net flux resulting from changes in cell growth. 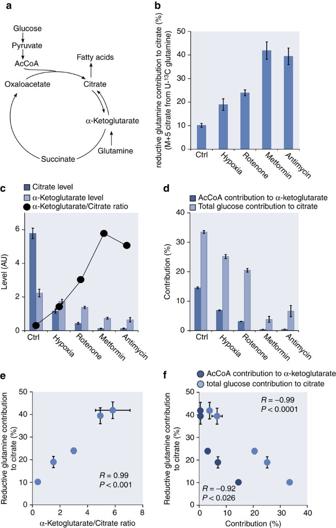Figure 1: Reductive carboxylation correlates with concomitant metabolic parameters. (a) Reductive (α-ketoglutarate to citrate) versus oxidative (citrate to α-ketoglutarate) flux and concomitant network reactions and metabolites. Reductive glutamine contribution to citrate (b), alterations in citrate and α-ketoglutarate levels (c) and AcCoA contribution to α-ketoglutarate (M+2 of α-ketoglutarate from U13C glucose), as well as total glucose contribution to citrate (d), for different stress conditions. Correlation between reductive glutamine contribution to citrate and the α-ketoglutarate to citrate ratio (e), and AcCoA contribution to α-ketoglutarate as well as total glucose contribution to citrate (f), Ctrl denotes standard culture condition. All error bars indicate the s.d. AllP-values (Student’st-test, two-tailed, unequal variance) and error bars are calculated from two independent replicates. Figure 1: Reductive carboxylation correlates with concomitant metabolic parameters. ( a ) Reductive (α-ketoglutarate to citrate) versus oxidative (citrate to α-ketoglutarate) flux and concomitant network reactions and metabolites. Reductive glutamine contribution to citrate ( b ), alterations in citrate and α-ketoglutarate levels ( c ) and AcCoA contribution to α-ketoglutarate (M+2 of α-ketoglutarate from U 13 C glucose), as well as total glucose contribution to citrate ( d ), for different stress conditions. Correlation between reductive glutamine contribution to citrate and the α-ketoglutarate to citrate ratio ( e ), and AcCoA contribution to α-ketoglutarate as well as total glucose contribution to citrate ( f ), Ctrl denotes standard culture condition. All error bars indicate the s.d. All P -values (Student’s t -test, two-tailed, unequal variance) and error bars are calculated from two independent replicates. Full size image Reductive carboxylation is regulated on a metabolic level To elucidate the mechanism responsible for the switch from oxidative to reductive glutamine utilization, we measured reductive glutamine contribution to citrate and changes in the levels of citrate and α-ketoglutarate using U- 13 C glutamine and gas chromatography–mass spectrometry [5] . We compared cells under conditions previously described to induce reductive glutamine metabolism: hypoxia, or treatment with rotenone, metformin and antimycin a [5] , [6] , [7] , [8] . The respiratory chain inhibitors rotenone, metformin and antimycin a were all used at concentrations that cause an ~50% decrease in oxygen consumption ( Supplementary Fig. S1 ). As expected, reductive glutamine contribution to citrate (identified by the level of the M+5 mass isotopomer of citrate from U- 13 C glutamine ( Supplementary Fig. S2a )) increased for all conditions compared with the control condition ( Fig. 1b ). Furthermore, the citrate and α-ketoglutarate levels decreased in all conditions; however, the decrease in citrate was much greater than the decrease in α-ketoglutarate ( Fig. 1c ). Strikingly, the α-ketoglutarate/citrate ratio correlated with the magnitude of reductive glutamine contribution to citrate ( Fig. 1b,c,e and Supplementary Data 1 ). This suggests that changes in the α-ketoglutarate/citrate ratio could be the principal driving force for the switch from oxidative glucose to reductive glutamine metabolism, promoting the use of glutamine as the primary carbon source for citrate synthesis. As lipogenic AcCoA is derived from citrate [5] , this ratio might determine the source of carbon for lipid synthesis ( Fig. 1a ). The correlation between reductive glutamine contribution to citrate and increased α-ketoglutarate/citrate ratio raises the question of how this ratio is determined. Besides glutamine, glucose can also contribute to citrate and α-ketoglutarate levels [17] . We inferred the latter flux contribution with a U- 13 C glucose tracer by measuring the total glucose contribution to citrate or the AcCoA contribution to α-ketoglutarate. Total glucose contribution to citrate and AcCoA contribution to α-ketoglutarate (M+2 of α-ketoglutarate from U- 13 C glucose ( Supplementary Fig. S2b )) decreased in all conditions compared to with control ( Fig. 1d ). Moreover, the percent of M+2 α-ketoglutarate from U- 13 C glucose and the percent citrate labelling from glucose both correlated inversely with the reductive glutamine contribution to citrate ( Fig. 1b,d,f ), and thus the α-ketoglutarate/citrate ratio ( Fig. 1c,d ). This suggests that carbon entry into the TCA cycle via AcCoA can affect the α-ketoglutarate/citrate ratio, and also suggest this as one point of regulation. If carbon entry into the TCA cycle via AcCoA regulates the α-ketoglutarate/citrate ratio and reductive glutamine contribution to citrate, then replenishing the pyruvate-derived citrate pool by forcing carbon into the TCA cycle via AcCoA should decrease reductive glutamine utilization. Increased glucose concentrations cannot be used to increase the oxidative carbon entry into the TCA cycle. However, as glucose can be converted to lactate, supplementing the media with high concentrations of lactate can impair cytosolic NAD + regeneration and promote increased carbon contribution via AcCoA into the TCA cycle. Addition of lactate to the culture media shifts the reaction direction of lactate dehydrogenase from net synthesis to net consumption of lactate to produce pyruvate [18] . As the pyruvate-to-lactate conversion is a major route of NAD + regeneration from NADH, higher lactate levels increase cytosolic NADH levels preventing cytosolic NAD + recovery and increase carbon contribution into the TCA cycle via AcCoA [19] ( Fig. 2a ). Moreover, lactate addition uncouples the use of glucose-derived carbon, as both lactate and glucose feed into the same pyruvate pool. Lactate supplementation in the control condition increased the AcCoA contribution to α-ketoglutarate (M+3 in α-ketoglutarate from U- 13 C glutamine ( Supplementary Fig. S2a )) and decreased the α-ketoglutarate/citrate ratio along with reductive glutamine contribution to citrate ( Supplementary Fig. S3a ). We confirmed that the increase in AcCoA contribution to α-ketoglutarate during lactate supplementation is a result of increased pyruvate entry by comparing M+3 in α-ketoglutarate from U- 13 C glutamine to M+2 in α-ketoglutarate, from U- 13 C lactate and U- 13 C glucose. We found that the sum of the M+2 contributions from glucose and lactate matched the M+3 contribution from glutamine, showing that supplementation of lactate leads to a joint contribution of glucose and lactate to pyruvate, and it’s entry into the AcCoA pool ( Supplementary Fig. S3b (left panel)). Subsequently, we applied lactate supplementation to conditions that induce reductive glutamine utilization and found that AcCoA contribution to α-ketoglutarate increased ( Fig. 2b ) and the α-ketoglutarate/citrate ratio decreased along with reductive glutamine contribution to citrate ( Fig. 2c, d and Supplementary Data 1 ). We again confirmed using the rotenone+lactate condition that both glucose and lactate contribute to the AcCoA pool ( Supplementary Fig. S3b (right panel)). Notably, the effect seen following exposure to hypoxia, rotenone and metformin was much more pronounced than that seen for antimycin a. This may be because of the fact that complex I inhibition can be circumvented using the glycerol phosphate shuttle to pass electrons to complex II, whereas a block in complex III cannot be bypassed [20] . Together, these data show that carbon conversion to citrate via AcCoA modulates the α-ketoglutarate/citrate ratio, which in turn might determine the reductive glutamine contribution to citrate. 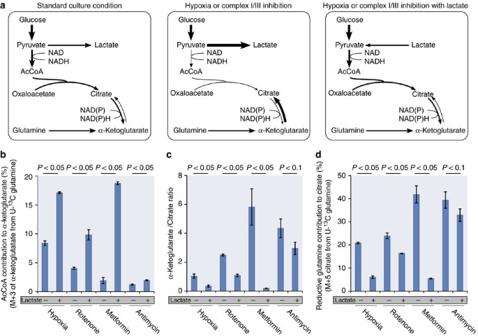Figure 2: Metabolic parameters modulate reductive carboxylation. (a) Lactate supplementation (25 mmol l−1) in the media prohibits glucose conversion to lactate and thus forces an increased glucose contribution to the TCA cycle. Flux and metabolite state in standard growth condition (left), hypoxia or complex I/III inhibition (middle), and hypoxia or complex I/III inhibition with lactate (right). Thickness of the arrows and the size of the metabolites indicates the magnitude of alteration. AcCoA contribution to α-ketoglutarate (calculated from a U-13C glutamine tracer: M+3 from glutamine is highly correlated with M+2 from glucose in A549:R=0.998,P=0.0001) (b), α-ketoglutarate/citrate ratio (c) and reductive glutamine contribution to citrate (d) for different stress conditions with and without lactate supplementation. All error bars indicate the s.d. AllP-values (Student’st-test, two-tailed, unequal variance) and error bars are calculated from two independent replicates. Figure 2: Metabolic parameters modulate reductive carboxylation. ( a ) Lactate supplementation (25 mmol l −1 ) in the media prohibits glucose conversion to lactate and thus forces an increased glucose contribution to the TCA cycle. Flux and metabolite state in standard growth condition (left), hypoxia or complex I/III inhibition (middle), and hypoxia or complex I/III inhibition with lactate (right). Thickness of the arrows and the size of the metabolites indicates the magnitude of alteration. AcCoA contribution to α-ketoglutarate (calculated from a U- 13 C glutamine tracer: M+3 from glutamine is highly correlated with M+2 from glucose in A549: R =0.998, P =0.0001) ( b ), α-ketoglutarate/citrate ratio ( c ) and reductive glutamine contribution to citrate ( d ) for different stress conditions with and without lactate supplementation. All error bars indicate the s.d. All P -values (Student’s t -test, two-tailed, unequal variance) and error bars are calculated from two independent replicates. Full size image To further test the hypothesis that the α-ketoglutarate/citrate ratio determines whether glutamine is converted oxidatively (via glutamine anaplerosis) or reductively (via reductive carboxylation), we reasoned that supplementing cells that have increased reductive glutamine usage with acetate (to directly replenish the citrate pool ( Fig. 3a )) or citrate should shift the ratio from reductive back to oxidative glutamine utilization. To test this possibility, we added acetate (25 mmol l −1 ) or citrate (0.3 and 1.2 mmol l −1 ) to cells in the presence of metformin. In the presence of acetate, we measured the α-ketoglutarate/citrate ratio and reductive glutamine contribution to citrate normalized to the total glutamine contribution to citrate with a U- 13 C glutamine tracer ( Supplementary Fig. S2a ). This normalization was undertaken to prevent the unlikely possibility that addition of acetate will disturb globally the metabolite pool sizes and thus lead to an overall decrease in glutamine contribution to the metabolites. Acetate decreased the α-ketoglutarate/citrate ratio and similarly reduced the normalized reductive glutamine contribution to citrate ( Fig. 3b,c ). The addition of acetate also led to increased oxidative glutamine metabolism in the TCA cycle ( Fig. 3d ). Furthermore, we tested whether acetate supplementation to metformin treatment also decreases the reductive glutamine contribution to palmitate using 5- 13 C glutamine ( Fig. 3e and Supplementary Fig. S4 ). In line with the citrate labelling data, we measured reduced 5- 13 C glutamine labelling in m+5 to m+8 palmitate when acetate is supplemented in the medium of metformin-treated cells. This finding corroborates that the reductive conversion of glutamine is reduced when acetate is added. With citrate supplementation, we measured the ratio between oxidative and reductive glutamine utilization using a U- 13 C-glutamine tracer. Measuring the α-ketoglutarate/citrate ratio in this condition is not possible because of residual media citrate impeding accurate measurements of intracellular citrate levels. We determined the ratio of oxidative versus reductive glutamine utilization based on M+4 in fumarate, malate and aspartate (oxidative contribution) and M+3 in fumarate, malate and aspartate (reductive contribution) ( Supplementary Fig. S2c ). We found that the ratio between oxidative and reductive glutamine utilization in the presence of metformin increased with increasing citrate concentrations ( Fig. 3f ), further arguing that the switch from oxidative to reductive glutamine utilization is a function of the α-ketoglutarate/citrate ratio. 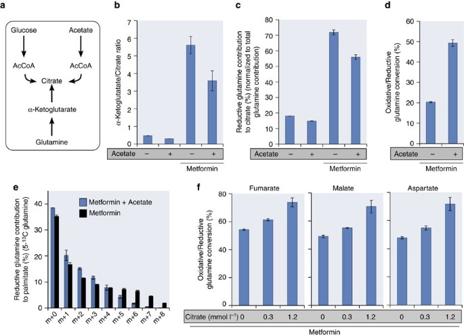Figure 3: The α-ketoglutarate/citrate ratio determines reductive glutamine utilization. (a) Acetate is a third carbon source beside glucose and glutamine that fuels the citrate pool. (b) α-Ketoglutarate/citrate ratio and (c) reductive glutamine contribution to citrate normalized to the total glutamine contribution to citrate, with and without acetate supplementation in the control condition and in the presence of metformin. (d) Ratio of oxidative versus reductive glutamine utilization in the presence of metformin with and without acetate measured with a U13C-glutamine tracer. (e) Glutamine contribution to palmitate in metformin treatment conditions with and without acetate supplementation. (f) Ratio of oxidative versus reductive glutamine utilization in the presence of metformin with and without different concentrations of citrate measured with a U13C-glutamine tracer determined from fumarate, malate and asparate. All error bars indicate the s.d.P-values are <0.05. AllP-values (Student’st-test, two-tailed, unequal variance) and error bars are calculated from two independent replicates. Figure 3: The α-ketoglutarate/citrate ratio determines reductive glutamine utilization. ( a ) Acetate is a third carbon source beside glucose and glutamine that fuels the citrate pool. ( b ) α-Ketoglutarate/citrate ratio and ( c ) reductive glutamine contribution to citrate normalized to the total glutamine contribution to citrate, with and without acetate supplementation in the control condition and in the presence of metformin. ( d ) Ratio of oxidative versus reductive glutamine utilization in the presence of metformin with and without acetate measured with a U 13 C-glutamine tracer. ( e ) Glutamine contribution to palmitate in metformin treatment conditions with and without acetate supplementation. ( f ) Ratio of oxidative versus reductive glutamine utilization in the presence of metformin with and without different concentrations of citrate measured with a U 13 C-glutamine tracer determined from fumarate, malate and asparate. All error bars indicate the s.d. P -values are <0.05. All P -values (Student’s t -test, two-tailed, unequal variance) and error bars are calculated from two independent replicates. Full size image To determine whether glucose contribution to the TCA cycle and the α-ketoglutarate/citrate ratio determines oxidative versus reductive glutamine metabolism in another cell line, we measured glucose contribution to the TCA cycle along with the corresponding α-ketoglutarate/citrate ratios under nine different growth conditions in 143B osteosarcoma cells. Analysis of U- 13 C glucose and U- 13 C glutamine tracer data demonstrates that the levels of reductive glutamine contribution to citrate varied by eightfold with treatments ( Fig. 4a and Supplementary Data 1 ). Addition of lactate, β-nicotinamide mononucleotide (NMN) (NAD + precursor) and the mitochondrial uncoupling agent carbonyl cyanide 4-(trifluoromethoxy)phenylhydrazone (FCCP) decreased reductive glutamine contribution, whereas addition of 5-aminoimidazole-4-carboxamide 1-β-D-ribofuranoside (AICAR) (a precursor of AMP) had only minor effects that were not statistically significant. Oligomycin (a direct inhibitor of mitochondrial ATP synthase), rotenone, metformin and antimycin a, all led to increased reductive glutamine contribution to citrate ( Fig. 4a ). The AcCoA contribution to α-ketoglutarate, the total pyruvate contribution to citrate, citrate, as well as the α-ketoglutarate/citrate ratio were correlated with reductive glutamine contribution to citrate ( Fig. 4b–h ). With the exception of lactate supplementation, total pyruvate contribution to citrate is given based on the total glucose contribution to citrate. In the case of lactate, the total pyruvate contribution to citrate is resembled by the sum of the total glucose and lactate contribution to citrate. Notably, for some stress conditions (lactate, oligomycin, rotenone and metformin), α-ketoglutarate instead of citrate is the major contributor to the change in the α-ketoglutarate/citrate ratio ( Fig. 4d ). Nonetheless, the α-ketoglutarate/citrate ratio, but not α-ketoglutarate or citrate levels themselves, correlate most strongly with the per cent reductive glutamine contribution to citrate ( Fig. 4g,h ). This observation strongly argues that the ratio, rather than the α-ketoglutarate nor the citrate concentration themselves, is the major determinant of reductive glutamine utilization. Thus, it is unlikely that α-ketoglutarate (or isocitrate) concentrations per se regulates isocitrate dehydrogenase on the enzyme level. 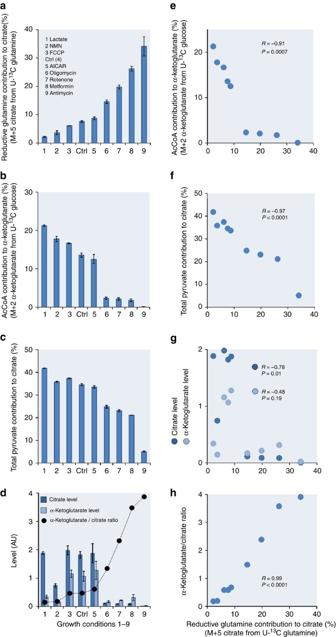Figure 4: Reductively derived citrate correlates with metabolic parameters in 143B cells. (a) Reductive glutamine contribution to citrate. (b) AcCoA contribution to α-ketoglutarate. (c) Total pyruvate contribution to citrate. (d) Alterations in citrate and α-ketoglutarate levels. Correlation between the reductive glutamine contribution to citrate and (e) the AcCoA contribution to α-ketoglutarate, (f) the total pyruvate contribution to citrate, (g) the relative citrate and α-ketoglutarate levels, and (h) the α-ketoglutarate/citrate ratio. In case of lactate supplementation, M+3 in α-ketoglutarate from U-13C glutamine instead of M+2 in α-ketoglutarate from U-13C glucose was used. Ctrl denotes standard culture condition. All error bars indicate the s.d. The correlation criteria wereR>0.7 orR<−0.7 andP<0.05. AllP-values (Student’st-test, two-tailed, unequal variance) and error bars are calculated from two independent replicates. Figure 4: Reductively derived citrate correlates with metabolic parameters in 143B cells. ( a ) Reductive glutamine contribution to citrate. ( b ) AcCoA contribution to α-ketoglutarate. ( c ) Total pyruvate contribution to citrate. ( d ) Alterations in citrate and α-ketoglutarate levels. Correlation between the reductive glutamine contribution to citrate and ( e ) the AcCoA contribution to α-ketoglutarate, ( f ) the total pyruvate contribution to citrate, ( g ) the relative citrate and α-ketoglutarate levels, and ( h ) the α-ketoglutarate/citrate ratio. In case of lactate supplementation, M+3 in α-ketoglutarate from U- 13 C glutamine instead of M+2 in α-ketoglutarate from U- 13 C glucose was used. Ctrl denotes standard culture condition. All error bars indicate the s.d. The correlation criteria were R >0.7 or R <−0.7 and P <0.05. All P -values (Student’s t -test, two-tailed, unequal variance) and error bars are calculated from two independent replicates. Full size image To expand our findings and exclude the possibility that the effects we observed could all be accounted for by an increase in α-ketoglutarate-to-citrate carbon exchange or be compromised by labelled CO 2 fixation, we measured the reductive glutamine contribution to the fatty acid palmitate in the PC3 prostate adenocarcinoma cell line ( Fig. 5 and Supplementary Data 1 ). Reductive glutamine contribution to palmitate was measured using a 5- 13 C-glutamine tracer, which reaches palmitate only through reductive glutamine metabolism ( Supplementary Fig. S4 ). The contribution of this tracer to palmitate was calculated based on an isotopic spectral analysis model [21] , [22] . The nine conditions tested spanned a 14-fold range of reductive glutamine contribution to palmitate ( Fig. 5 ). Similar to the results obtained with citrate labelling in A549 and 143B cells, reductive glutamine contribution to palmitate correlated with AcCoA contribution to α-ketoglutarate, the total glucose contribution to citrate and the α-ketoglutarate/citrate ratio ( Fig. 5 ). These results further corroborate the hypothesis that the above mentioned criteria determine the extent of reductive glutamine metabolism across a wide range of cellular conditions. 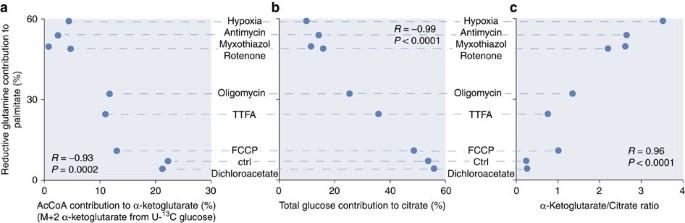Figure 5: Reductively derived fatty acids correlate with metabolic parameters in PC3 cells. Correlation between the reductive glutamine contribution to fatty acids (palmitate) and (a) the AcCoA contribution to α-ketoglutarate, (b) the total glucose contribution to citrate and (c) the α-ketoglutarate/citrate ratio. Ctrl denotes standard culture condition. AllP-values are calculated with Student’st-test (two-tailed, unequal variance). Figure 5: Reductively derived fatty acids correlate with metabolic parameters in PC3 cells. Correlation between the reductive glutamine contribution to fatty acids (palmitate) and ( a ) the AcCoA contribution to α-ketoglutarate, ( b ) the total glucose contribution to citrate and ( c ) the α-ketoglutarate/citrate ratio. Ctrl denotes standard culture condition. All P -values are calculated with Student’s t -test (two-tailed, unequal variance). Full size image To further elucidate that an increase in reductive glutamine contribution to citrate results in a net flux increase such as it has been shown previously for hypoxia [5] , we measured the net reductive glutamine flux to palmitate in the presence of antimycin a, oligomycin or 2-thenoyltrifluoroacetone (TTFA) ( Supplementary Fig. S5 ). In accordance with results observed under hypoxia, we found that the net reductive glutamine flux to palmitate increased in the presence of antimycin a, oligomycin or TTFA by approximately six-, five- and threefold, respectively ( Supplementary Fig. S5 ). This data suggests that at least in certain conditions this major switch in carbon fueling results also in a net flux increase. Multiple upstream events influence carbon entry into the TCA cycle To investigate whether there is a sole signalling event that controls carbon entry into the TCA cycle via AcCoA, we further tested how reductive glutamine contribution to citrate is regulated under hypoxia and in the presence of complex I/III inhibitors (rotenone, metformin and antimycin a). It has been shown previously that inhibition of PDK1 with dichloroacetate (DCA) reduces the contribution of reductive glutamine carboxylation in hypoxia [5] . To evaluate the extent by which PDKs impact reductive glutamine utilization, we determined the effect of the PDK inhibitor DCA [23] , [24] on the reductive glutamine contribution to citrate in the presence of rotenone, metformin or antimycin a. The dose of DCA was adjusted to a concentration that significantly reduced pyruvate dehydrogenase (PDH) E1a Ser232 phosphorylation in hypoxia ( Supplementary Fig. S6 ). The concentration of 5 mmol l −1 DCA that met these criteria matches the concentration used previously [5] . Our data corroborated that PDK inhibition by DCA significantly reduced reductive glutamine contribution to citrate in hypoxia ( Fig. 6a ) [5] , but DCA did not alter reductive carboxylation in the presence of complex I/III inhibitors ( Fig. 6a ), suggesting that these stresses may utilize distinct mechanisms. 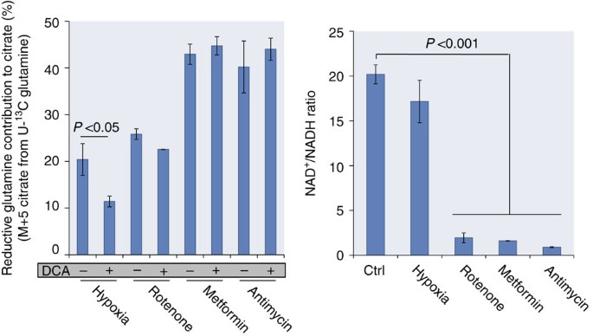Figure 6: PDK1 regulates carbon entry into the TCA cycle in hypoxia. (a) Reductive glutamine contribution to citrate for different stress conditions with and without the PDK inhibitor DCA. (b) NAD+/NADH ratio for different stress conditions. Ctrl denotes standard culture condition. All error bars indicate the s.d. AllP-values (Student’st-test, two-tailed, unequal variance) and error bars are calculated from three independent replicates. Figure 6: PDK1 regulates carbon entry into the TCA cycle in hypoxia. ( a ) Reductive glutamine contribution to citrate for different stress conditions with and without the PDK inhibitor DCA. ( b ) NAD + /NADH ratio for different stress conditions. Ctrl denotes standard culture condition. All error bars indicate the s.d. All P -values (Student’s t -test, two-tailed, unequal variance) and error bars are calculated from three independent replicates. Full size image One consequence of respiratory chain inhibition is decreased mitochondrial conversion of NADH to NAD + and thus a reduced mitochondrial NAD + /NADH ratio [6] , [25] . Interestingly, the pyruvate dehydrogenase reaction is coupled to this cofactor ratio [17] ; therefore, it is possible that changes in the mitochondrial NAD + /NADH ratio following complex I/III inhibition are responsible for reduced carbon entry into the TCA cycle via AcCoA. To test this hypothesis, we measured the NAD + /NADH ratio using HPLC ( Supplementary Fig. S8 ), in cells growing in standard culture conditions and under the four stress conditions. We confirmed literature data that, indeed, the NAD + /NADH ratio decreased by more than tenfold in the presence of complex I/III inhibitors compared with that of the control ( Fig. 6b ); however, there was no significant alteration of the NAD + /NADH ratio under hypoxia ( Fig. 6b ). We further estimated from the lactate to pyruvate ratio the amount of free NAD + /NADH in the cytosol. As expected, the cytosolic lactate to pyruvate ratio [26] increased following rotenone, metformin and antimycin a treatment ( Supplementary Fig. S9 ), suggesting that the total decrease in NAD + /NADH measured likely occurs mainly in the mitochondria. Thus, this ratio could mediate the directionality of glutamine metabolism in the presence of respiratory chain inhibitors. To test whether the lower NAD + /NADH ratio limits carbon entry into the TCA cycle during respiratory chain inhibition and to exclude a bias because of the fact that we can directly measure only total but not free NAD + /NADH, we supplemented the media with the NAD + precursor NMN. Supplementation of cells with NMN increases the free NAD + level [27] , thus increasing the NAD + /NADH ratio ( Fig. 7a ). As expected from literature data, NMN addition increased the NAD + /NADH ratio in the presence of metformin by more than fivefold compared with the presence of metformin alone ( Fig. 7b ). Moreover, the AcCoA contribution to α-ketoglutarate increased when NMN was added to metformin-treated cells, while the reductive glutamine contribution decreased ( Fig. 7c,d ). These data suggest that changes in the NAD + /NADH ratio elicited by respiratory chain inhibitors changes the α-ketoglutarate/citrate ratio, which in turn shifts glutamine utilization from oxidative to reductive. 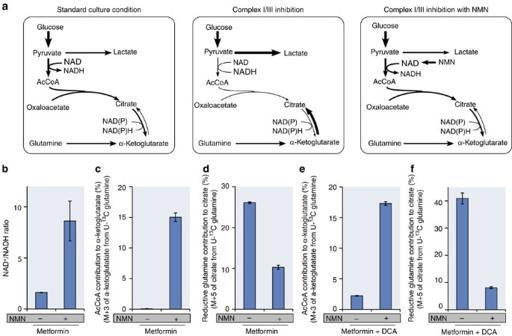Figure 7: NAD+/NADH ratio limits carbon entry into the TCA cycle. (a) NMN supplementation (25 mmol l−1) increased NAD+level and thus increased the NAD+/NADH ratio, which leads to increased glucose flux through pyruvate dehydrogenase. Flux and metabolite state in standard growth condition (left), hypoxia or complex I/III inhibition (middle) and hypoxia or complex I/III inhibition with NMN (right). Thickness of the arrows and the size of the metabolites indicate the magnitude of alteration. NAD+/NADH ratio (b), AcCoA contribution to α-ketoglutarate (c) and reductive glutamine contribution to citrate (d) in the presence of metformin with and without NMN supplementation. AcCoA contribution to α-ketoglutarate (e) and reductive glutamine contribution to citrate (f) in the presence of metformin and PDK inhibitor DCA with and without NMN supplementation. All error bars indicate the s.d.P-values between with and without NMN supplementation are <0.05. AllP-values (Student’st-test, two-tailed, unequal variance) and error bars are calculated from two independent replicates. Figure 7: NAD + /NADH ratio limits carbon entry into the TCA cycle. ( a ) NMN supplementation (25 mmol l −1 ) increased NAD + level and thus increased the NAD + /NADH ratio, which leads to increased glucose flux through pyruvate dehydrogenase. Flux and metabolite state in standard growth condition (left), hypoxia or complex I/III inhibition (middle) and hypoxia or complex I/III inhibition with NMN (right). Thickness of the arrows and the size of the metabolites indicate the magnitude of alteration. NAD + /NADH ratio ( b ), AcCoA contribution to α-ketoglutarate ( c ) and reductive glutamine contribution to citrate ( d ) in the presence of metformin with and without NMN supplementation. AcCoA contribution to α-ketoglutarate ( e ) and reductive glutamine contribution to citrate ( f ) in the presence of metformin and PDK inhibitor DCA with and without NMN supplementation. All error bars indicate the s.d. P -values between with and without NMN supplementation are <0.05. All P -values (Student’s t -test, two-tailed, unequal variance) and error bars are calculated from two independent replicates. Full size image Although the above data suggest that the NAD + /NADH ratio affects the pyruvate dehydrogenase reaction, it is unclear whether this happens directly via cofactor coupling or indirectly via effects on PDK4 activity. Thus, we tested whether PDK4 is expressed differently in hypoxia compared with the complex I/III inhibitors ( Supplementary Fig. S3c ). We found that the PDK4 expression increased by approximately threefold during metformin treatment compared with hypoxia. PDK4-mediated phosphorylation inhibits pyruvate dehydrogenase activity and PDK4 is known to be strongly regulated by the NAD + /NADH ratio [28] . If the pyruvate dehydrogenase complex is directly inhibited by the NAD + /NADH ratio via cofactor coupling, instead of PDK4-mediated phosphorylation, addition of NMN in the presence of DCA (which inhibits PDK4 (ref. 28 )) and metformin should still increase the AcCoA contribution to α-ketoglutarate ( Fig. 7a ). Thus, we added DCA at concentrations determined to block PDHE1a phosphorylation ( Supplementary Fig. S6 ) and found that NMN increased AcCoA contribution to α-ketoglutarate and, as expected, decreased reductive glutamine contribution to citrate in the presence of metformin plus DCA, excluding the involvement of PDK4 ( Fig. 7e,f ). Although the NAD + /NADH ratio can control carbon entry into the TCA cycle, and thus reductive carboxylation, other regulatory events resulting from complex I/III inhibition cannot be excluded. These data suggest that although alterations in PDH activity via phosphorylation can promote reductive carboxylation, this is not the only mechanism active under all conditions. Reductive glutamine contribution to metabolites and biomass building blocks was recently identified as a phenomenon to support growth of hypoxic and respiratory chain impaired cells [5] , [6] , [7] , [8] . We demonstrate here a general mechanistic explanation for how metabolic rearrangements enable reductive glutamine contribution to citrate ( Fig. 8 ). Although our approach is limited in looking at cell metabolite levels without information about compartmentalization of pathways, with the consequence that we cannot provide thermodynamic calculations, we identified the α-ketoglutarate/citrate ratio itself as a critical determinant of reductive glutamine utilization. In some cases, this may not represent a true increase in net flux, but a relative flux change with increased exchange may also be involved as both lead to increased 5-carbon-labelled citrate from glutamine. Nevertheless, altered α-ketoglutarate/citrate ratios can promote increased net reductive glutamine flux under some conditions including hypoxia [5] or treatment with antimycin a, oligomycin or TTFA. 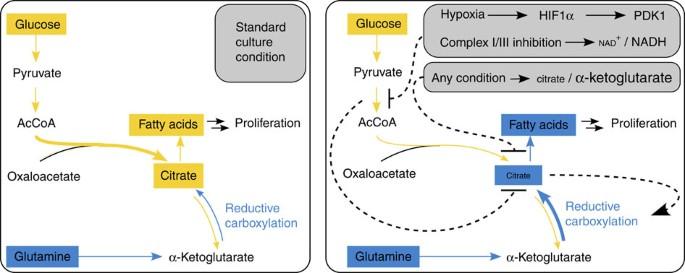Figure 8: Reductive glutamine carboxylation is a function of the α-ketoglutarate to citrate ratio. In standard growth conditions, proliferation-relevant fatty acids are produced mainly from glucose (left). Any stress condition leading to an increased α-ketoglutarate to citrate ratio alters glutamine conversion from oxidative to reductive (right). Subsequently, proliferation-relevant fatty acids are produced mainly from glutamine (right). Dashed lines indicate the regulatory flow. Size of the metabolites and arrow thickness indicate the magnitude of alteration. Figure 8: Reductive glutamine carboxylation is a function of the α-ketoglutarate to citrate ratio. In standard growth conditions, proliferation-relevant fatty acids are produced mainly from glucose (left). Any stress condition leading to an increased α-ketoglutarate to citrate ratio alters glutamine conversion from oxidative to reductive (right). Subsequently, proliferation-relevant fatty acids are produced mainly from glutamine (right). Dashed lines indicate the regulatory flow. Size of the metabolites and arrow thickness indicate the magnitude of alteration. Full size image A wide range of conditions influence the α-ketoglutarate/citrate ratio by modulating carbon entry into the TCA cycle via AcCoA. Moreover, our data demonstrate that other events (for example, acetate or citrate supplementation) that alter the α-ketoglutarate/citrate ratio will have a role in determining whether glutamine is metabolized oxidatively or reductively. Regarding the carbon entry into the TCA cycle via AcCoA, there are at least two upstream mechanisms explaining how carbon entry (and subsequent downstream metabolic changes) are regulated. In the case of hypoxia, decreased carbon entry into the TCA cycle is driven at least in part by PDK1-mediated inhibition of pyruvate dehydrogenase, whereas complex I/III inhibition decreases carbon entry into the TCA cycle through a decrease in the NAD + /NADH ratio. The latter is the result of mitochondrial electron transport inhibition, which in turn decreases pyruvate to AcCoA conversion likely via cofactor coupling. By extension, any condition that affects the α-ketoglutarate/citrate ratio, regardless of the upstream regulation that initiates this change, is predicted to alter reductive versus oxidative glutamine utilization and consequently the fueling source for proliferation relevant fatty acid synthesis. Although our approach has the limitation that we cannot conclude whether reductive carboxylation takes place in the mitochondria or the cytosol, this mechanistic understanding allows for the first time predictions of environmental and genetic conditions, which promote reductive glutamine utilization and might lead to the development of drugs inhibiting this process. Although reductive carboxylation has mainly been investigated in cancer cells, there is evidence that at least some non-transformed cell also use this pathway (for example, non-transformed cells from brown fat (differentiated brown adipocytes [22] ), lung (MRC5 (ref. 5 )), prostate (p69; S.-M. Fendt, unpublished data) and normal lymphocytes [5] Hence, this mode of regulation may allow carbon metabolism to rapidly adapt to changing growth conditions. In this way, the cell can immediately switch carbon source utilization without involving complex transcriptional or allosteric regulation and ensure optimal substrate usage to support growth under various conditions. Furthermore, this mechanism is a consequence of any upstream event altering α-ketoglutarate and/or citrate levels and requires no further energy investment. Yet, to which extent NAD(P) + /NAD(P)H levels, which are cofactors coupled to the α-ketoglutarate to citrate ratio and affect the activity of enzymes, such as glutamate dehydrogenase, influence the reaction direction remains to be determined, but some influence is likely based on kinetic considerations. As a result, targeting reductive glutamine metabolism for therapeutic benefit may require an approach that impacts intrinsic properties of the metabolic network, rather than interruption of signalling events that indirectly influence the process. Cell lines and cell culture conditions All cell lines were obtained from ATCC. All experiments were performed in DMEM (Mediatech) with 10% dialysed fetal bovine serum (Invitrogen) and 1% pen/strep (Mediatech), and glucose or glutamine with either U- 13 C glucose (CLM-1396 Cambridge Isotopes), U- 13 C glutamine (605166 Sigma) or 5- 13 C glutamine (CLM-1166 Cambridge Isotopes). Cell lines were treated for 1 day or, in case of fatty acid labelling, for 3 days. Growth conditions were altered in the following ways: AICAR 0.25 mmol l −1 (143B), antimycin 2 μg ml −1 (PC3) and 20 ng l −1 (A549, 143B), citrate 0.3 and 1.2 mmol l −1 (A549), DCA 5 mmol l −1 (A549, PC3), FCCP 10 μmol l −1 (PC3) and 2.5 μmol l −1 (143B), hypoxia 1% (A549, 143B, PC3), lactate 25 mmol l −1 (A549, 143B), metformin 1 mmol l −1 (A549, 143B), myxothiazol 1 μmol l −1 (PC3), NMN 25 mmol l −1 (A549, 143B), oligomycin 5 μmol l −1 (PC3) and 2.5 μmol l −1 (143B), rotenone 1 μg ml −1 (PC3) and 10 ng ml −1 (A549, 143B) and TTFA 400 μmol l −1 (PC3). All compounds were obtained from Sigma. Oxygen consumption Oxygen consumption was measured with an Oxytherm instrument (Hansatech). Cells were trypsinized and resuspended in fresh media. Oxygen consumption of detached cells was measured for 10 min. The slope of the linear range was used to calculate rates. Error bars are from biological replicates. Carbon contribution to TCA cycle and palmitate To assess metabolite levels and metabolite labelling, we applied the methods described in Metallo et al. [5] In brief, labelled tissue cultures were washed with saline and metabolism was quenched with −20 °C cold 65% methanol. After cell scraping in 65% methanol, −20 °C cold chloroform was added and the samples were vortexed at 4 °C to extract metabolites. Phase separation was achieved by centrifugation at 4 °C. Methanol phase (polar metabolites) and chloroform phase (fatty acids) were separated and dried by applying constant air flow. Dried metabolite samples were stored at −80 °C. Polar metabolite samples were derivatized with methoxyamine (Thermo Scientific) for 90 min at 40 °C and subsequently with N -(tert-butyldimethylsilyl)- N -methyl-trifluoroacetamide, with 1% tert-Butyldimethylchlorosilane (Sigma) for 60 min at 60 °C. Fatty acids were esterified with sulphuric acid/methanol for 120 min at 60 °C and subsequently extracted with hexane. Isotopomer distributions of polar metabolites and fatty acids were measured with a 6890N GC system (Agilent Technologies) combined with a 5975B Inert XL MS system (Agilent Technologies). One microlitre of samples was injected in splitless mode with an inlet temperature of 270 °C onto a DB35MS column. The carrier gas was helium with a flow rate of 1 ml min −1 . For the measurement of polar metabolites the oven was held at 100 °C for 3 min and then ramped to 300 °C with a gradient of 2.5 °C min −1 . For fatty acid samples, the oven was held at 80 °C for 1 min and ramped with 5 °C min −1 to 300 °C. The MS system was operated under electron impact ionization at 70 eV. A mass range of 100–650 amu was scanned. Isotopomer distributions were extracted from the raw ion chromatograms using a custom Matlab M-file, which applies consistent integration bounds and baseline correction to each ion [29] . In addition, we corrected for naturally occurring isotopes using the method of Fernandez et al. [30] Total contribution of carbon was calculated using the following equation [31] : Here n is the number of C atoms in the metabolite, i the different mass isotopomers and m the abundance of a certain mass. In the case of lactate supplement, total pyruvate contribution instead of total glucose contribution is depicted and M+3 of α-ketoglutarate from U- 13 C glutamine was used as a measure for AcCoA contribution to α-ketoglutarate. For relative metabolite levels, the total ion count was normalized to the internal standard norvaline and to cell number counted with an automated cell counter (Nexcelom). Isotopomer distributions of fatty acids were further fitted to an isotopic spectral analysis model previously described [5] . Isotopic spectral analysis is a non-linear regression method for fitting the gas chromatography–mass spectrometry data to a model for biosynthesis with two unknowns, D , the fractional contribution of the labelled precursor to the biosynthetic precursor pool, and g ( t ), the fraction of newly synthesized product present at time t [21] , [22] . During citrate supplementation, we specifically focus on the ratio between oxidative and reductive glutamine conversion, because absolute contributions cannot be inferred because of variations in the label dilution at different amounts of supplementation. Moreover, high concentrations of unlabelled and residual citrate from the media prevented the accurate measurement of label in this pool; hence, the ratio of oxidative versus reductive glutamine utilization was determined from the measurement of M+4 in fumarate, malate and aspartate (oxidative contribution) and M+3 in fumarate, malate and aspartate (reductive contribution) ( Supplementary Fig. S2c ). The net reductive glutamine fluxes to palmitate in the presence or absence of antimycine, oligomycine or TTFA were calculated as described by Metallo et al. [5] , based on the fractional contribution of reductively utilized glutamine and the fraction of newly synthesized glutamine ( D and g ( t ) from the isotopic spectral analysis model) combined with cell numbers and growth rates [5] . Raw data are depicted in Supplementary Data 1 . Error bars are from biological replicates. We verified for our data set that glutaminolysis, protein turnover and CO2 refixation can be neglected. This is necessary because glutamiolysis can occur in mammalian cells [32] and CO2 refixation has been shown to be important in microbes [33] . Therefore, we analysed M+0 from pyruvate on a U- 13 C glutamine tracer (significantly altered M+0 indicates glutaminolysis), M+5 of glutamine from a U- 13 C glutamine tracer (significantly altered M+5 indicates protein turnover), and M+1 and M+2 from a 1- 13 C glutamine tracer (M+2 indicates CO2 refixation) ( Supplementary Fig. S7 ). In accordance with previous reports [5] , [34] , [35] , we found that glutaminolysis, protein turnover and CO2 refixation can be neglected. NAD + /NADH ratio The protocol used to extract NAD+/NADH from cells was adapted from a previously described method [36] . In brief, tissue culture cells were washed with ice-cold PBS and immediately quenched with liquid nitrogen. Cold extraction solution (−20 °C; 40% methanol, 40% acetonitrile, 20% buffer) was added and plates were incubated at −20 °C for 15 min. Cells were scraped on dry ice and centrifuged at 4 °C. The supernatant was collected and the remaining pellet re-extracted twice with extraction solution. The supernatant was dried and analysed by high-pressure liquid chromatography. The quenching protocol was validated by measuring the ATP, ADP and AMP with liquid chromatography–mass spectrometry. The calculated energy charge was 0.73. Dried extracts were dissolved in water and separation of compounds was achieved by HPLC using an Agilent (C8) 2.6 × 250 mm, 5 μmol l −1 particle column (Agilent Technologies). The HPLC method was adapted from a published method [37] and verified. Mobile phase flow rate was 1 ml min −1 . Eluent A (50 mmol l −1 potassium phosphate dibasic and 8 mmol l −1 tetrabutylammonium bisulphate aqueous adjusted to pH 5.8) and eluent B (50 mmol l −1 potassium phosphate dibasic and 8 mmol l −1 tetrabutylammonium bisulphate aqueous solution adjusted to pH 5.8 with 40% acetonitrile) were applied with a time-dependent gradient. Absorbance of NAD was detected at 254 nm wavelength and NADH was detected at 254 nm and 340 nm. The method was verified with calibration curves, which are depicted in Supplementary Fig. S8 . Error bars are from biological replicates. Western blot PDH and phospo-PDH antibodies were obtained from Invitrogen or Calbiochem, respectively, and were diluted to 1 or 0.25 μg ml −1 , respectively. Statistics Error bars depict s.d. R and P -values for the depicted correlations were calculated with the Matlab integrated function corrcoef: [R,P]=corrcoef returns P , a matrix of P -values for testing the hypothesis of no correlation. Each P -value is the probability of getting a correlation as large as the observed value by random chance, when the true correlation is zero. P -values were also calculated for bar graphs using a Student’s t -test (two-tailed, unequal variance) to determine whether two samples are likely to have come from the same two underlying populations that have the same mean. How to cite this article: Fendt, S.-M. et al. Reductive glutamine metabolism is a function of the α-ketoglutarate to citrate ratio in cells. Nat. Commun. 4:2236 doi: 10.1038/ncomms3236 (2013).